Infrared light excites cells by changing their electrical capacitance Optical stimulation has enabled important advances in the study of brain function and other biological processes, and holds promise for medical applications ranging from hearing restoration to cardiac pace making. In particular, pulsed laser stimulation using infrared wavelengths >1.5 μm has therapeutic potential based on its ability to directly stimulate nerves and muscles without any genetic or chemical pre-treatment. However, the mechanism of infrared stimulation has been a mystery, hindering its path to the clinic. Here we show that infrared light excites cells through a novel, highly general electrostatic mechanism. Infrared pulses are absorbed by water, producing a rapid local increase in temperature. This heating reversibly alters the electrical capacitance of the plasma membrane, depolarizing the target cell. This mechanism is fully reversible and requires only the most basic properties of cell membranes. Our findings underscore the generality of pulsed infrared stimulation and its medical potential. Optical technologies that enable precise local perturbation of nerve or muscle activity play an increasingly important role in neuroscience and the development of treatments for neurological, psychiatric and cardiovascular disease. Most such technologies require the target tissue to be sensitized using a light-sensitive gene (for example, channelrhodopsin) [1] , [2] or chemical (for example, caged neurotransmitters) [3] , [4] , adding technical complexity and risk to their applications, especially in the clinical setting. In contrast, pulsed infrared laser light has been shown to stimulate neural and other excitable cells in vivo without any genetic or chemical pre-treatment [5] . Most of the radiation wavelengths used for these studies ( λ =1470–1550 nm and λ =1840–2120 nm) can be delivered via an optical fibre, providing flexibility for minimally invasive delivery. Infrared stimulation targets have included peripheral and cranial motor nerves [6] , [7] , cavernous nerves in the prostate [8] , vestibular hair cells [9] , the cochlear nerve [10] and the heart [11] . The simplicity of direct infrared excitation makes it attractive for a variety of basic and clinical applications ranging from hearing restoration to cardiac pace making [12] . Despite mounting evidence from animal studies that infrared stimulation can be used to modulate biological function, its underlying mechanism(s) are unknown. It has been shown that infrared stimulation is accompanied by rapid increases in tissue temperature [13] , which has been speculated to excite cells by affecting ion channel gating, activating intracellular second messengers, forming membrane pores, triggering thermosensitive ion channels or otherwise increasing membrane conductance [12] , [13] , [14] . No direct evidence has been put forth for any of these putative mechanisms. In part, this may reflect the fact that most experiments with infrared stimulation to date have relied on downstream read-outs of its effect (for example, action potential (AP) generation and muscle contraction) rather than directly assaying target cells through electrophysiology. We investigated the mechanism of infrared stimulation in Xenopus laevis oocytes, cultured mammalian cells and artificial lipid bilayers, and identified an unexpected general mechanism whereby infrared laser pulses absorbed by water produce a rapid local increase in temperature, which transiently increases membrane electrical capacitance, thus generating depolarizing currents. This finding has important implications for infrared stimulation of the nervous system and other organs, and raises questions about the effects of other forms of optical energy on cell signalling. Infrared light elicits depolarizing currents in untreated oocytes The large size of X. laevis oocytes ( ∼ 1 mm) enables simultaneous electrophysiological recording and optical stimulation of the cell with minimal potential for light-electrode artifacts (such as changes in seal or pipet resistance). Based on previous results indicating that infrared radiation increases cell excitability [13] , [14] , we first applied infrared laser pulses to oocytes expressing voltage-gated sodium (Na + ) or potassium (K + ) channels, searching for specific changes in their open probability upon irradiation. Contrary to expectations, we saw infrared effects that were independent of the type of expressed channels, and in fact were the same in wild-type oocytes as they were in oocytes expressing the ion channels. Consequently, we report here our results from wild-type oocytes. 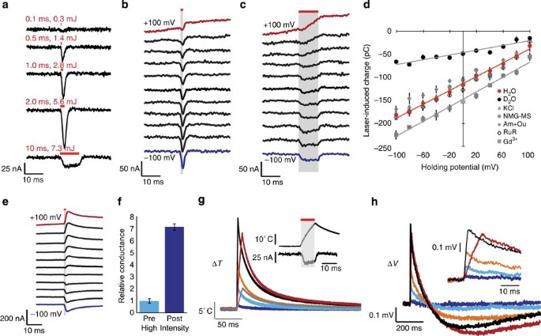Figure 1: Infrared laser pulses evoke inward currents in wild-type oocytes via a water-heating mechanism. (a) Currents recorded in voltage-clamped oocytes held at −80 mV evoked by infrared laser pulses of 0.1 ms (0.3 mJ) to 10 ms (7.3 mJ) duration and energy. Red lines above each trace indicate when the pulse was applied. (b) I–V response to the application of a 1 ms (2.8 mJ) pulse. (c) I–V response to the application of a 10 ms (7.3 mJ) pulse. (d) Q–V curves acquired in H2O-based SOS solution (H2O), D2O-based SOS solution (D2O), SOS solution in which NaCl has been replaced by KCl (KCl), SOS solution in which NaCl has been replaced byN-methyl-D-glucamine–methanesulphonate (NMG–MS), and SOS solution supplemented with 1 mM amiloride and 1 mM oubain (Am+Ou), 250 μM ruthenium red (RuR) or 1 mM GdCl3(Gd3+).N=5 for each measurement. Where they are not visible, error bars (s.e.m.) are smaller than the corresponding symbols. Linear fits are shown for the H2O, D2O and Gd3+data to aid in their comparison. (e) I–V response to a 1 ms (2.8 mJ) pulse after the oocyte has been exposed to pulses of energy >8 mJ. I–V responses were recorded at equally spaced voltages from −100 to +100 mV. Traces are spaced and coloured for clarity. The red bar and grey shading indicate the timing of laser stimulation. (f) Relative conductance (normalized sum of current magnitudes at holding potentials of −80 and +40 mV) of voltage-clamped oocytes before and after stimulation with pulses >8 mJ.N=5. (g) Local temperature responses acquired using calibrated pipet resistance to infrared pulses of 0.1 ms (0.3 mJ) (blue), 0.5 ms (1.4 mJ) (cyan), 1 ms per 2.8 mJ (orange), 2 ms (5.6 mJ) (black) and 10 ms (7.3 mJ) (red). The grey trace shows temperature response to a 10 ms (7.3 mJ) pulse in D2O solution. The insert shows a comparison of temperature response and current recording to a 10 ms (7.3 mJ) pulse. (h) Voltage responses recorded in current-clamped oocytes stimulated with the same set of pulses (similarly colour-denoted as in (g)). The resting potentials were −46±4.6 mV. The insert shows a zoomed-in view of the first 30 ms following the start of the laser pulse. All error bars are ±s.e.m. Figure 1a shows that stimulation of wild-type oocytes with infrared laser pulses of 100 μs to 10 ms duration (pulse energies of 0.28 mJ to 7.3 mJ) elicited inward currents under voltage-clamp conditions. Current duration and amplitude corresponded to laser pulse width and energy. Infrared pulses lasting 10 ms, substantially longer than the voltage-clamp response time, allowed the natural shape of the current response to be resolved; a square-shaped current began with the onset of the laser pulse and ended immediately after the laser was turned off. Currents were inward at holding potentials from −100 mV to +100 mV ( Fig. 1b,c ) with a linear charge–voltage (QV) response reversing at an extrapolated 140±18 mV ( Fig. 1d ). Maximal current amplitudes of 86±5.4 nA were observed with 2 ms (5.6 mJ) pulses. With an optical fibre diameter of 400 μm and a penetration depth in water of <200 μm for 1889 nm light [15] , only ∼ 5% of the oocyte surface area is stimulated by infrared pulses. Stimulating an entire oocyte would thus be expected to elicit currents of up to 1.7 μA. Figure 1: Infrared laser pulses evoke inward currents in wild-type oocytes via a water-heating mechanism. ( a ) Currents recorded in voltage-clamped oocytes held at −80 mV evoked by infrared laser pulses of 0.1 ms (0.3 mJ) to 10 ms (7.3 mJ) duration and energy. Red lines above each trace indicate when the pulse was applied. ( b ) I–V response to the application of a 1 ms (2.8 mJ) pulse. ( c ) I–V response to the application of a 10 ms (7.3 mJ) pulse. ( d ) Q–V curves acquired in H 2 O-based SOS solution (H 2 O), D 2 O-based SOS solution (D 2 O), SOS solution in which NaCl has been replaced by KCl (KCl), SOS solution in which NaCl has been replaced by N -methyl- D -glucamine–methanesulphonate (NMG–MS), and SOS solution supplemented with 1 mM amiloride and 1 mM oubain (Am+Ou), 250 μM ruthenium red (RuR) or 1 mM GdCl 3 (Gd 3+ ). N =5 for each measurement. Where they are not visible, error bars (s.e.m.) are smaller than the corresponding symbols. Linear fits are shown for the H 2 O, D 2 O and Gd 3+ data to aid in their comparison. ( e ) I–V response to a 1 ms (2.8 mJ) pulse after the oocyte has been exposed to pulses of energy >8 mJ. I–V responses were recorded at equally spaced voltages from −100 to +100 mV. Traces are spaced and coloured for clarity. The red bar and grey shading indicate the timing of laser stimulation. ( f ) Relative conductance (normalized sum of current magnitudes at holding potentials of −80 and +40 mV) of voltage-clamped oocytes before and after stimulation with pulses >8 mJ. N =5. ( g ) Local temperature responses acquired using calibrated pipet resistance to infrared pulses of 0.1 ms (0.3 mJ) (blue), 0.5 ms (1.4 mJ) (cyan), 1 ms per 2.8 mJ (orange), 2 ms (5.6 mJ) (black) and 10 ms (7.3 mJ) (red). The grey trace shows temperature response to a 10 ms (7.3 mJ) pulse in D 2 O solution. The insert shows a comparison of temperature response and current recording to a 10 ms (7.3 mJ) pulse. ( h ) Voltage responses recorded in current-clamped oocytes stimulated with the same set of pulses (similarly colour-denoted as in ( g )). The resting potentials were −46±4.6 mV. The insert shows a zoomed-in view of the first 30 ms following the start of the laser pulse. All error bars are ±s.e.m. Full size image With pulse energies <8 mJ, stimulation elicited a consistent, transient current response over hundreds of trials. However, a few pulses at radiant energies exceeding 8 mJ were sufficient to irreversibly alter the oocyte's response to infrared. Subsequent to this energy barrier being breached, even lower-energy pulses produced a longer-lasting current reversing close to 0 mV ( Fig. 1e ). High-energy stimulation also tended to make oocytes more leaky ( Fig. 1f ). Presumably, this irreversible high-energy effect represents a form of damage to the oocyte membrane (indeed, local discolouration was sometimes seen on the oocyte surface after the experiment) and we did not investigate it further, confining pulse energies for the rest of our study to <8 mJ. The large positive reversal potential for infrared-induced currents suggested an ionic conductance selective for Na + or calcium (Ca 2+ ). However, we found that current magnitudes and reversal potentials were not significantly affected by eliminating channel-permeable ions from extracellular solution (using N -methyl- D -glucamine as a cation and methanesulphonate as anion) or replacing Na + with K + in the physiological recording buffer ( Fig. 1d ). Responses were also not significantly affected by ion channel and transporter inhibitors ruthenium red, ouabain and amiloride. Gadolinium (Gd 3+ ) was observed to shift the apparent reversal potential further in the positive direction rather than inhibiting the current. It has previously been suggested that water is the primary chromophore responsible for absorbing infrared light and converting it into energy for cell excitation [13] . At 1889 nm, H 2 O has an absorption coefficient of 60.6 cm −1 (ref. 15 ). The absorption coefficient for heavy water (D 2 O) is approximately fivefold lower at this wavelength [16] . Replacing H 2 O with D 2 O in the extracellular recording solution produced a 65.3±4.1% decrease in response to infrared laser pulses, confirming the role of water in the excitation mechanism ( Fig. 1d ). We measured the time course of local infrared-induced temperature changes in aqueous buffer using calibrated pipet resistance [17] . Laser pulses produced roughly linear increases in temperature of up to 22.2±0.6°C (for a 7.3 mJ pulse), followed by a decay to baseline with a time constant of ∼ 100 ms ( Fig. 1g ), matching the heat relaxation time for water. In D 2 O solution, temperature changes were reduced by about 70% ( Fig. 1g ). Comparing the time course of the temperature change to the oocyte current elicited by infrared reveals that oocyte currents correspond more closely to the rate of change in solution temperature than to the absolute temperature. In current-clamp mode, infrared pulses depolarized oocytes from their resting potential by 0.6±0.03 mV (5.6 mJ pulse, Fig. 1h ). The resting potential was recovered within 500ms, followed by an overshoot hyperpolarization of ∼ 40% of the depolarization magnitude. Adjusting for the 5% fractional stimulation of the oocyte, a depolarization of 11–12 mV would be expected for full-cell excitation. Infrared light elicits depolarizing currents in mammalian cells To determine whether the infrared-induced currents observed in oocytes were unique to that preparation, we performed infrared stimulation experiments in whole-cell-clamped HEK cells. Laser pulses of 200 μs (0.7 mJ) and 1 ms (3.7 mJ) elicited current responses similar to those seen in oocytes ( Fig. 2a,b ). Maximal current amplitudes of 73±20 pA were observed with 1 ms pulses. Currents were inward at all potentials examined, with an apparent reversal at 146±10.8 mV. 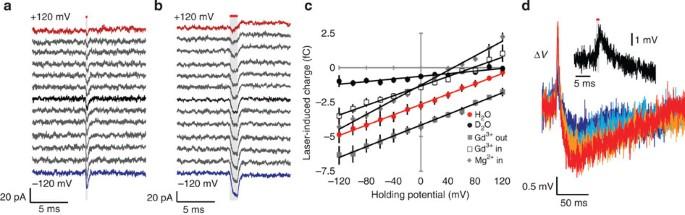Figure 2: Infrared evokes inward currents in untransfected HEK cells. (a) I–V response in voltage-clamped HEK293T cells to the application of a 0.2 ms (0.7 mJ) pulse. (b) I–V response to a 1 ms (3.7 mJ) pulse. I–V responses were recorded at equally spaced voltages from −120 to +120 mV. Traces are spaced and coloured for clarity. The red bar and grey shading indicate the timing of laser stimulation. (c) Q–V curves acquired in HEK cells with H2O-based recording solutions (H2O), D2O-based bath solution (D2O), with 1 mM GdCl3added to bath solution (Gd3+out), 1 mM GdCl3added to pipet solution (Gd3+in) or 20 mM MgCl2added to pipet solution with 0 mM MgCl2in the bath (Mg2+in).N=5 for each measurement. Error bars are ±s.e.m. Data are fitted with lines to aid in their comparison. (d) Voltage responses recorded in current-clamped HEK cells with 0.5 ms (1.9 mJ) (blue), 1 ms (3.7 mJ) (cyan), 1.5 ms (5.6 mJ) (orange) and 2 ms (7.4 mJ) (red) pulses. Insert provides a zoomed-in view of the first 30 ms following the start of a 1-ms pulse. Figure 2: Infrared evokes inward currents in untransfected HEK cells. ( a ) I–V response in voltage-clamped HEK293T cells to the application of a 0.2 ms (0.7 mJ) pulse. ( b ) I–V response to a 1 ms (3.7 mJ) pulse. I–V responses were recorded at equally spaced voltages from −120 to +120 mV. Traces are spaced and coloured for clarity. The red bar and grey shading indicate the timing of laser stimulation. ( c ) Q–V curves acquired in HEK cells with H 2 O-based recording solutions (H 2 O), D 2 O-based bath solution (D 2 O), with 1 mM GdCl 3 added to bath solution (Gd 3+ out), 1 mM GdCl 3 added to pipet solution (Gd 3+ in) or 20 mM MgCl 2 added to pipet solution with 0 mM MgCl 2 in the bath (Mg 2+ in). N =5 for each measurement. Error bars are ±s.e.m. Data are fitted with lines to aid in their comparison. ( d ) Voltage responses recorded in current-clamped HEK cells with 0.5 ms (1.9 mJ) (blue), 1 ms (3.7 mJ) (cyan), 1.5 ms (5.6 mJ) (orange) and 2 ms (7.4 mJ) (red) pulses. Insert provides a zoomed-in view of the first 30 ms following the start of a 1-ms pulse. Full size image Owing to the small size of HEK cells relative to the optical fibre diameter and light penetration depth, both the cell and the recording pipet were irradiated by light pulses. Infrared pulses applied directly to a pipet tip reduce pipet resistance, and may also reduce seal resistance. These effects were observed to confound QV curves measured with pulse energies >2.8 mJ ( Supplementary Fig. S1 ). Thus 0.7 mJ pulses were used for QV analysis. Replacing the H 2 O in extracellular solution with D 2 O reduced the observed current response in HEK cells by 75.8±12.6% ( Fig. 2c ). Similar to oocytes, extracellular application of GdCl 3 produced a positive shift in the reversal potential. Applying GdCl 3 in the intracellular solution produced the opposite effect. Increasing the concentration of magnesium chloride (MgCl 2 ) in the pipet solution also negatively shifted the reversal potential ( Fig. 2c ). In current-clamp mode, infrared light depolarized cells by up to 2.7 mV (1ms, 3.7-mJ pulse, Fig. 2d ). The extent of depolarization appeared to saturate with longer pulses in the 0.5–2 ms range, potentially due to concomitant changes in pipet, seal or membrane resistance. Our measurement may therefore underestimate the change in membrane potential one would obtain in unpatched cells. Undershooting repolarization similar to that seen in oocytes was observed after the initial response. Infrared light changes the capacitance of artificial bilayers Our observation of infrared-induced currents in untreated oocytes and HEK cells, and their failure to respond to channel and transporter blockers, led us to consider a general membrane-related mechanism. In particular, we noted that the time course of the current response to infrared pulses tracks the rate of change in temperature and not the temperature itself ( Fig. 1g ). This led us to hypothesize that temperature alters the electrical capacitance of the membrane, producing a current proportional to the derivative of capacitance, and thereby to the derivative of temperature, with respect to time. We tested this possibility in artificial lipid bilayers, which are a good minimal model of living membranes because they have no proteins and minimal membrane conductance compared with cells. We tested the effects of infrared pulses on voltage-clamped bilayers prepared from 1:1 phosphatidylcholine (PC) and phosphatidylethanolamine (PE). Infrared pulses elicited currents of up to 406±44 pA (1 ms, 2.8 mJ), which reversed, notably, near 0 mV ( Fig. 3a–c ). The shape of the observed current was similar to those seen in oocytes and HEK cells. Replacing H 2 O with D 2 O in the recording buffer reduced the response by 79.3±12.6% ( Fig. 3c ). 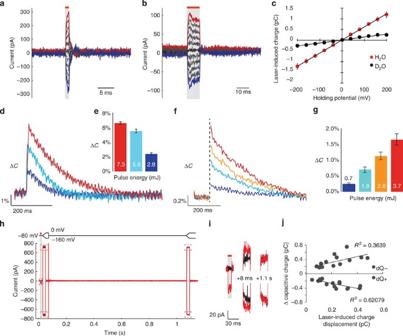Figure 3: Infrared transiently alters the membrane electrical capacitance of artificial lipid bilayers and HEK cells. (a) I–V current response in voltage-clamped artificial lipid bilayer comprising (1:1) PE:PC (PC:PE) in symmetric NaCl solution to 1 ms (2.8 mJ) infrared pulse. (b) I–V current response in voltage-clamped PE:PC bilayer in symmetric NaCl solution to 10 ms (7.3 mJ) infrared pulse. Traces are coloured for clarity. The red bar and grey shading indicate the timing of laser stimulation. Voltages ranged from −200 to +200 mV. (c) Q–V curves acquired in PE:PC lipid bilayers in response to 10 ms (7.3 mJ) infrared stimulation in H2O-based (H2O) and D2O-based (D2O) symmetric NaCl solution.N=5 for each measurement. (d) Changes in membrane electrical capacitance in a PE:PC bilayer induced by 1 ms (2.8 mJ) (purple), 2 ms (5.6 mJ) (cyan), and 10 ms (7.3 mJ) (red) infrared pulses, determined from current responses to a sinusoidal voltage input. (e) Maximum changes in equivalent capacitance at each pulse energy (N=5). (f) Changes in membrane equivalent capacitance in HEK cells induced by 0.2 ms (0.7 mJ) (purple), 0.5 ms (1.9 mJ) (cyan), 0.75 ms (2.8 mJ) (orange) and 1 ms (3.7 mJ) (red) infrared pulses determined from current responses to dual-sinusoidal voltage input. (g) Maximum changes in equivalent capacitance in HEK cells at each pulse energy (N=5). (h) Current responses of a PE:PC bilayer to voltage-clamp protocol (shown above current traces) starting with a holding potential at −80 mV, ramping to 0 or −160 mV, stepping back to −80 mV and ramping again to 0 or −160 mV after 1.1 s. In black traces, no infrared light is applied. In red traces, a 10 ms (7.3 mJ) infrared pulse is applied before the first ramp. Red traces are overlaid on black ones; four total traces are shown. (i) Zoomed view of the five boxed areas of (h), in the same relative spatial arrangement as they appear in (h). (j) Comparison of change in capacitive charge (integral of the difference between red and black traces in the first current ramp) and laser-induced charge displacement in individual traces collected using the paradigm of panel (h) using infrared pulse energies of 2.3–7.3 mJ. All error bars are ±s.e.m. In panelsa,b,handithe red lines and grey shading indicate the timing of infrared laser pulse. Figure 3: Infrared transiently alters the membrane electrical capacitance of artificial lipid bilayers and HEK cells. ( a ) I–V current response in voltage-clamped artificial lipid bilayer comprising (1:1) PE:PC (PC:PE) in symmetric NaCl solution to 1 ms (2.8 mJ) infrared pulse. ( b ) I–V current response in voltage-clamped PE:PC bilayer in symmetric NaCl solution to 10 ms (7.3 mJ) infrared pulse. Traces are coloured for clarity. The red bar and grey shading indicate the timing of laser stimulation. Voltages ranged from −200 to +200 mV. ( c ) Q–V curves acquired in PE:PC lipid bilayers in response to 10 ms (7.3 mJ) infrared stimulation in H 2 O-based (H 2 O) and D 2 O-based (D 2 O) symmetric NaCl solution. N =5 for each measurement. ( d ) Changes in membrane electrical capacitance in a PE:PC bilayer induced by 1 ms (2.8 mJ) (purple), 2 ms (5.6 mJ) (cyan), and 10 ms (7.3 mJ) (red) infrared pulses, determined from current responses to a sinusoidal voltage input. ( e ) Maximum changes in equivalent capacitance at each pulse energy ( N =5). ( f ) Changes in membrane equivalent capacitance in HEK cells induced by 0.2 ms (0.7 mJ) (purple), 0.5 ms (1.9 mJ) (cyan), 0.75 ms (2.8 mJ) (orange) and 1 ms (3.7 mJ) (red) infrared pulses determined from current responses to dual-sinusoidal voltage input. ( g ) Maximum changes in equivalent capacitance in HEK cells at each pulse energy ( N =5). ( h ) Current responses of a PE:PC bilayer to voltage-clamp protocol (shown above current traces) starting with a holding potential at −80 mV, ramping to 0 or −160 mV, stepping back to −80 mV and ramping again to 0 or −160 mV after 1.1 s. In black traces, no infrared light is applied. In red traces, a 10 ms (7.3 mJ) infrared pulse is applied before the first ramp. Red traces are overlaid on black ones; four total traces are shown. ( i ) Zoomed view of the five boxed areas of ( h ), in the same relative spatial arrangement as they appear in ( h ). ( j ) Comparison of change in capacitive charge (integral of the difference between red and black traces in the first current ramp) and laser-induced charge displacement in individual traces collected using the paradigm of panel ( h ) using infrared pulse energies of 2.3–7.3 mJ. All error bars are ±s.e.m. In panels a , b , h and i the red lines and grey shading indicate the timing of infrared laser pulse. Full size image If the infrared-induced temperature jumps causes an increase in membrane capacitance, such an increase would be expected to persist after the initial laser-induced current, with a decay time resembling that of the absolute temperature of the bilayer and surrounding solution. We used a sinusoidal voltage-clamp paradigm [18] to directly measure changes in bilayer electrical capacitance. Our measurements revealed infrared-induced increases in capacitance of up to 6.6±0.2% (7.3 mJ pulse) that decayed on a timescale of 100–200 ms ( Fig. 3d,e ), consistent with the rate of thermal relaxation. Infrared-induced changes in membrane capacitance were similarly measured in HEK cells in the whole-cell configuration. Infrared dose-dependent increases in membrane capacitance of up to 1.6±0.2% (3.7 mJ pulse) were observed ( Fig. 3f,g ). Capacitance increases decay on a timescale of ∼ 200 ms. To further illustrate the relationship between laser-induced currents and changes in membrane capacitance, we designed a voltage-clamp protocol in which voltage ramps were applied to bilayers 8 ms and 1.1 s after an infrared pulse. Increases in ramp current magnitude relative to control were seen in both positive and negative directions immediately after the laser pulse, but are absent in ramps applied 1.1 s later ( Fig. 3h,i ). The magnitude of such increases was correlated with the magnitude of laser-induced charge displacement ( Fig. 3j ). Capacitive effect is consistent with classical theory The total electrical capacitance of a lipid membrane in electrolyte solution reflects a combination of the core capacitance of the phospholipid bilayer and the in-series capacitance of ionic double layers on each side of the membrane [19] . This total capacitance can be modelled using the Gouy–Chapman–Stern (GCS) theory of double layer capacitors [20] . This textbook theory, derived from the Poisson equation, models a charged surface in contact with electrolyte solution. Taking into account the relevant dielectric constants and ionic composition, GCS calculates the electrical capacitance of the system by balancing the electrical and thermal forces affecting the spatial distribution of ions near the charged surface. Although this classical theory has well-known limitations [21] , it is a useful starting point from which to understand the capacitance changes observed in our experiments. We used the GCS model to simulate currents arising from temperature-dependent capacitance changes (illustrated by the equivalent circuit in Fig. 4a and Supplementary Fig. S2 ). Using the coupled equations (1) and (2) below (modified from Genet et al . [22] ), we solved numerically for surface potentials Φ o and (Φ i − V m ) on each side of the bilayer as a function of membrane potential and temperature. This allowed us to calculate net membrane capacitive charge. > It is noteworthy that temperature appears explicitly in two places in Eqs. (1) and (2) and implicitly in the temperature dependence of the aqueous dielectric permittivity ɛ T sol (ref. 23 ). Using this model, we simulated currents arising from infrared-induced temperature jumps (such as shown in Fig. 1g ). For a 1:1 PE:PC bilayer in symmetric monovalent electrolyte, the model predicts a current response time course similar to those we measured experimentally ( Fig. 4b,c ). A reasonable set of parameter values produced simulated current magnitudes within 25% of the measurement. 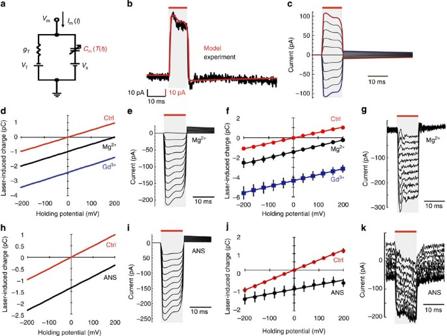Figure 4: Thermally induced changes in membrane electrical capacitance are consistent with capacitor theory. (a) Simplified equivalent circuit diagram and current equation for a passive membrane. The membrane current (Im(t)) depends on the membrane voltage (Vm), the Thevenin conductance (gT) and potential (VT), bilayer surface charges (represented byVs) and the temperature-dependent membrane capacitance (Cm(T(t))), highlighted in red. (b) Simulated current response (red) for a PE:PC bilayer in symmetric NaCl solution at a holding potential of +200 mV, based on the temporal profile of temperature response to a 10 ms (7.3 mJ) infrared pulse. An experimental current response for the same set of conditions is shown in black. (c) Simulated I–V response to a 10 ms (7.3 mJ) pulse at voltages ranging from −200 mV (blue) to +200 mV (red). (d) Q–V curves predicted by the model for PE:PC:PS bilayers with symmetric NaCl solution (Ctrl), and with 14 mM MgCl2(Mg2+) or 1 mM GdCl3(Gd3+) added to the 'outside' solution. (e) Simulated I–V response for the Mg2+condition in (d). (f) Q–V curves measured experimentally in solutions matching the conditions modelled in (d).N=5 per measurement. (g) Representative I–V response for the Mg2+condition in (f). (h) Q–V curves predicted by the model for PE:PC bilayers in symmetric NaCl solution (Ctrl) and with the 'outside' negative surface charge increased by 66% (ANS). (i) Simulated I–V response for the ANS condition in (h). (j) Q–V curves measured experimentally for PE:PC bilayers after (ANS) and before (Ctrl) the addition of 100 μM ANS.N=5 per measurement. (k) Representative I–V response corresponding to the ANS condition in (j). All I–V plots are for voltages ranging from −200 to +200 mV. In panelsb, c, e, g, iandkthe red bars and grey shading indicate the timing of the infrared laser pulse. All error bars infandjare ±s.e.m. Figure 4: Thermally induced changes in membrane electrical capacitance are consistent with capacitor theory. ( a ) Simplified equivalent circuit diagram and current equation for a passive membrane. The membrane current ( I m ( t )) depends on the membrane voltage ( V m ), the Thevenin conductance ( g T ) and potential ( V T ), bilayer surface charges (represented by V s ) and the temperature-dependent membrane capacitance ( C m (T(t))), highlighted in red. ( b ) Simulated current response (red) for a PE:PC bilayer in symmetric NaCl solution at a holding potential of +200 mV, based on the temporal profile of temperature response to a 10 ms (7.3 mJ) infrared pulse. An experimental current response for the same set of conditions is shown in black. ( c ) Simulated I–V response to a 10 ms (7.3 mJ) pulse at voltages ranging from −200 mV (blue) to +200 mV (red). ( d ) Q–V curves predicted by the model for PE:PC:PS bilayers with symmetric NaCl solution (Ctrl), and with 14 mM MgCl 2 (Mg 2+ ) or 1 mM GdCl 3 (Gd 3+ ) added to the 'outside' solution. ( e ) Simulated I–V response for the Mg 2+ condition in ( d ). ( f ) Q–V curves measured experimentally in solutions matching the conditions modelled in ( d ). N =5 per measurement. ( g ) Representative I–V response for the Mg 2+ condition in ( f ). ( h ) Q–V curves predicted by the model for PE:PC bilayers in symmetric NaCl solution (Ctrl) and with the 'outside' negative surface charge increased by 66% (ANS). ( i ) Simulated I–V response for the ANS condition in ( h ). ( j ) Q–V curves measured experimentally for PE:PC bilayers after (ANS) and before (Ctrl) the addition of 100 μM ANS. N =5 per measurement. ( k ) Representative I–V response corresponding to the ANS condition in ( j ). All I–V plots are for voltages ranging from −200 to +200 mV. In panels b, c, e, g, i and k the red bars and grey shading indicate the timing of the infrared laser pulse. All error bars in f and j are ±s.e.m. Full size image The model predicts a 0-mV reversal potential for infrared-induced currents when lipid surface charge and electrolyte composition are the same on both sides of the bilayer. However, this symmetry is predicted to be broken by placing multivalent cations on only one side of a symmetrically negatively charged bilayer, or by having an asymmetric surface charge. We modelled and experimentally tested scenarios ( Fig. 4d–g ) in which a symmetrically negatively charged lipid bilayer (1:1:1 PE:PC:PS (phosphatidylserine)) had MgCl 2 or GdCl 3 added to only the 'external' side of the membrane. Both model and experiment showed the reversal potential shifting positive. This model and artificial bilayer result is in agreement with our observations in oocytes and HEK cells, where adding multivalent cations Gd 3+ or Mg 2+ to one side of the membrane shifted the reversal potential so as to produce greater currents towards the other side ( Figs 1d , 2c ). We also modelled and experimentally tested a scenario in which the surface charge of a 1:1 PE:PC bilayer in symmetric buffer is made more negative on one side by adding the amphipathic anion 1-anilino-8-naphthalenesulphonate (ANS) to the external solution ( Fig. 4h–k ). Again, there was qualitative agreement between model and experiment for a positive shift in the reversal potential. Experiments with ANS are confounded by its gradual voltage-dependent permeation across the bilayer. This may partly explain the different shape of the infrared-induced current response in ANS-treated bilayers relative to theory and other experimental conditions. Infrared pulses depolarize bilayers by up to 9 mV Artificial bilayers are a good system in which to test infrared-induced changes in membrane potential. Unlike oocytes, most or all of the membrane is irradiated by the light; unlike HEK cells, the light does not irradiate a pipet electrode thereby introducing changes in circuit resistance. We made passive measurements of membrane potential in artificial bilayers under conditions where their positive reversal potential mimics those of oocytes and HEK cells (that is, PE:PC:PS with asymmetric MgCl 2 ). Infrared-induced depolarizations of up to 8.7±1.0 mV were observed ( Fig. 5a,b ). This magnitude of depolarization is consistent with the extrapolation of oocyte voltage changes to a condition in which the entire oocyte surface is stimulated (11–12 mV). Notably, the undershoot repolarization observed in oocytes and HEK cells was absent in artificial bilayers, which is consistent with a higher ratio of membrane capacitance to membrane conductance in bilayers as compared with oocytes and HEK cells, as illustrated by equivalent circuit simulations ( Supplementary Fig. S2 ). 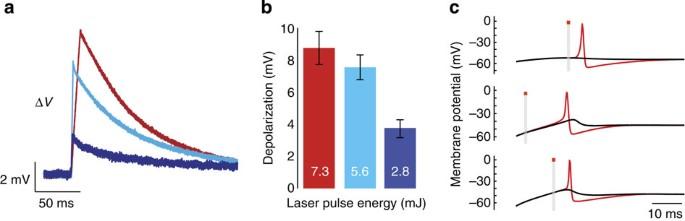Figure 5: Infrared depolarizes bilayers and elicits APs in artificial neurons. (a) Voltage responses in current-clamped artificial bilayers containing PE:PC:PS (PE:PC:PS) in NaCl solution, with 15 mM MgCl2added to the 'outside solution' (producing a reversal potential similar to that seen in oocytes and HEK cells). Responses were recorded for 1 ms (2.8 mJ) (blue), 2 ms per 5.6-mJ (cyan) and 10 ms (7.3 mJ) (red) pulses. (b) Maximum voltage responses to pulses with the indicated energies.N=3 per measurement. Error bars are ±s.e.m. (c) Voltage recordings from oocytes co-expressing voltage-gated sodium (Nav1.4 α,β) and potassium (Shaker) channels under loose voltage-clamp conditions, with (red) and without (black) a 1 ms (2.8 mJ) infrared laser pulse applied during a subthreshold voltage step. Red bars and grey shading indicate the timing of infrared laser pulse. Figure 5: Infrared depolarizes bilayers and elicits APs in artificial neurons. ( a ) Voltage responses in current-clamped artificial bilayers containing PE:PC:PS (PE:PC:PS) in NaCl solution, with 15 mM MgCl 2 added to the 'outside solution' (producing a reversal potential similar to that seen in oocytes and HEK cells). Responses were recorded for 1 ms (2.8 mJ) (blue), 2 ms per 5.6-mJ (cyan) and 10 ms (7.3 mJ) (red) pulses. ( b ) Maximum voltage responses to pulses with the indicated energies. N =3 per measurement. Error bars are ±s.e.m. ( c ) Voltage recordings from oocytes co-expressing voltage-gated sodium (Nav1.4 α,β) and potassium (Shaker) channels under loose voltage-clamp conditions, with (red) and without (black) a 1 ms (2.8 mJ) infrared laser pulse applied during a subthreshold voltage step. Red bars and grey shading indicate the timing of infrared laser pulse. Full size image Infrared light elicits APs Infrared stimulation has been shown in vivo to elicit APs and corresponding downstream effects in nerves. As neuronal cell bodies, processes and associated glia express a variety of proteins that could be involved in transducing infrared effects, we wanted to test the ability of infrared stimulation to elicit APs in a stripped-down 'artificial neuron'. Oocytes coexpressing voltage-gated sodium (Nav1.4 α,β) and potassium (Shaker) channels can fire APs when depolarized past threshold from a pre-pulse of −90 mV using a loose voltage clamp. When depolarized to potentials just below threshold, oocytes failed to fire APs. Under these conditions, a single infrared laser pulse of 1 ms (2.8 mJ) at or shortly before peak depolarization was sufficient to elicit an AP ( Fig. 5c ). For this effect to work, oocytes had to be within 0.5–1 mV of their firing threshold. As <5% of the oocyte surface is exposed to infrared light, preparations where the laser irradiates a larger fraction of membrane surface (such as neurons in vivo ) may permit infrared pulses to elicit APs from cells at membrane voltages much further below the threshold, as illustrated for a Hodgkin–Huxley model neuron in Supplementary Fig. S3 . The potential utility of infrared stimulation has been demonstrated by numerous in vivo studies, but the lack of understanding of its underlying mechanisms has hindered progress towards valuable scientific and clinical applications. In this study, we have uncovered an important and unexpected mechanism of infrared stimulation, mediated by transient changes in membrane electrical capacitance. Three model systems, oocytes, mammalian cells and artificial lipid bilayers, exhibited similar electrophysiological responses to infrared stimulation, with currents tracking the rate of change in temperature induced by the laser pulse. These currents were fully reversible and highly reproducible across specimens. When normalized by laser pulse energy, membrane voltage and approximate irradiated membrane area, infrared-induced charge displacement was similar between oocytes, HEK cells and artificial bilayers (1.9×10 −5 , 1.32×10 −5 and 0.9×10 −5 pC mJ −1 μm −2 , respectively). These data suggest that a common underlying mechanism is at work across these three systems, and that only the most basic elements of a cell membrane, represented by the artificial bilayer, are necessary for the infrared effect. Consistent with this conclusion, current responses in oocytes were unchanged when expressing voltage-gated channels, and were not abrogated by eliminating permeant ions or treating the oocytes with blockers of ion channels and transporters. Currents in all three systems were significantly reduced by replacing H 2 O with D 2 O, confirming directly for the first time that water is the major chromophore involved in infrared stimulation. The temporal profile of water-mediated temperature changes shows a rapid, near-linear rise during the laser pulse, followed by a slower exponential decay consistent with the heat relaxation time of water. We hypothesized that infrared-induced currents are produced by a transient change in membrane electrical capacitance upon local heating of the membrane and adjacent solution with the laser pulse. We obtained direct experimental evidence to support this hypothesis from bilayers and HEK cells, with the apparent membrane capacitance increasing by 6.6±0.2% (in bilayers) immediately after a (10 ms, 7.3 mJ) infrared pulse, and decaying to baseline on the timescale of 100–200 ms. The literature on optical stimulation of cells has largely overlooked the possibility of a capacitive mechanism [13] . However, a temperature-induced change in membrane capacitance is not surprising if one considers its underlying physics. The capacitance is established by ions whose spatial distribution near the membrane is determined by a balance of electrical and thermal forces. Thus, our implementation of the classical GCS theory of double layer capacitors generated predictions that largely corroborated our data in artificial bilayers. It also predicted ways to alter the reversal potential of infrared-induced currents (using multivalent ions or asymmetric changes in surface charge) that were effective in bilayers, HEK cells and oocytes. Our results are consistent with the early work on squid giant axons showing that higher temperatures led to increased membrane capacitance [24] , and the observation that light-induced temperature jumps in oocytes elicited charge displacement currents [25] . Our results do not exclude the possibility that other potential capacitance-modifying phenomena, such as changes in mechanical pressure, also have a role. Such potential contributions will require further study. What accounts for the positive reversal potential of infrared-induced currents in HEK cells and oocytes? In HEK cells, where it was possible to control solution contents on both sides of the membrane, the reversal potential was positive even with fully symmetric solutions. It is therefore likely that membrane factors such as differential surface charge, bilayer headgroup size, sugar modification, protein expression or some other factor besides solution contents are the primary drivers of positive reversal potential. For example, our model predicts a positive reversal potential when the outer leaflet of the membrane has a more negative surface charge or a thicker Stern layer than the inner leaflet. Intriguingly, both oocytes [26] and mammalian cells [27] are glycosylated on their outer surface, adding bulky groups with multivalent negative charges (however, their inner leaflets are thought to contain more negatively charged PS or phosphatidylinositol groups). Surface charge asymmetry is also necessary for normal ion channel function in excitable cells [28] . The generality of the capacitive mechanism for infrared stimulation is consistent with its documented ability to exert effects on a variety of cell types in vivo , including peripheral nerves, sensory ganglia and cardiac muscle cells [5] , [10] , [11] . The stimulus energies used in our study (0.28 –7.3 mJ) are similar to those used in vivo —either in single pulse mode or as trains of lower-energy pulses at repetition rates faster than aqueous thermal relaxation. In vivo results obtained from chilled nerves are also consistent with capacitive currents depending on temperature changes rather than temperature absolute values [13] . Blood perfusion in tissues is not expected to affect the dynamics of thermal laser stimulation [29] . In most cases, the consequence of successful nerve stimulation is an AP. Our demonstration that infrared stimulation could elicit APs in an 'artificial neuron' preparation expressing only voltage-gated sodium and potassium channels confirms that a capacitive mechanism can trigger cell firing when combined with a minimal set of AP machinery. Our model system had to be close to its firing threshold for infrared stimulation to trigger an AP, which is likely due to the fact that we stimulated <5% of the oocyte surface. A more completely stimulated preparation—artificial bilayers—exhibited potential changes of up to 9 mV with infrared stimulation, compared with <1 mV in oocytes. Thus, cells in vivo that are smaller than the stimulating fibre are expected to spike in response to infrared pulses from membrane potentials much further from their AP firing threshold. A neuron simulated using Hodgkin and Huxley (H&H) equations [28] exhibited robust generation of APs due to changes in capacitance of the type we measured experimentally. In vivo , cells whose membrane potentials are closer to threshold at the time of stimulation would be expected to have a greater likelihood of spiking. In fact, recent in vivo data suggest that cells costimulated electrically and optically show a greater response than with optical stimulation alone [30] . Biological mechanisms of depolarization, such as excitatory postsynaptic potentials, may have a similar effect. Neuronal response to infrared stimulation is expected to further depend on the channel composition of the cell, the cellular compartment being irradiated, and potentially features of its surrounding environment, such as myelination. Our circuit simulations suggest that cell depolarization induced by infrared pulses of various duration depends on membrane resistance; cells with lower resistance require infrared energy to be delivered by shorter pulses. Infrared-induced temperature increases should also affect the opening kinetics of voltage-dependent Na + and K + channels, whose relative concentration will determine the shape of the AP response to infrared stimulation. However, this rate constant effect is not expected to excite cells on its own, as demonstrated by our H&H simulation. Further studies are needed to more precisely characterize the capacitive mechanism of infrared stimulation and explore how its knowledge may enhance the use of this technology in vivo . For example, it would be interesting to model the effect of infrared on ion displacement at the molecular level and the resulting changes in local potentials experienced by voltage-gated Na + channels. Also, an understanding of the membrane properties of various cell types represented in vivo may help dissect which cells respond most strongly to infrared stimulation and mediate downstream physiological effects. Furthermore, it may be interesting to ask whether changes in cell membrane capacitance have a role when infrared, ultrasound or other forms of thermogenic energy are applied to other parts of the body. In the meantime, our finding that infrared stimulation produces its effect on cells by changing their membrane capacitance provides strong support for the use of this unique optical technology in biology and medicine. Pulse infrared laser stimulation Diode lasers (Capella and Renoir RINS, Aculight, Bothell, WA, USA) were used to stimulate cells and bilayers. These lasers emit infrared light centred at 1889 nm (for oocyte and bilayer recordings) or 1869 nm (for HEK cell recordings). Pulse durations (and corresponding energies) were set as stated in the text. For oocyte stimulation, a laser fibre with a diameter of 400 μm was positioned ∼ 100 μm below the oocyte resting on a quartz cover slip. For HEK cell stimulation, a 600-μm fibre was positioned inside the recording solution, within 500 μm of the cell, using a micromanipulator. A 400-μm or 200-μm fibre was similarly positioned in the recording solution in the top chamber of the artificial bilayer setup. Oocyte recordings X. laevis oocytes (stage IV–V, defolliculated, 1–3 days post surgery) were voltage- and current-clamped using a two-electrode setup (OC-725A, Warner Instruments, Hamden, CT, USA) using standard technique [31] . Glass recording pipets were used with initial bath resistance of 0.3–0.6 MΩ. Recordings were acquired with Innovative Integration DSP boards controlled by in-house written software and analysed using in-house software. Except where mentioned specifically, the oocytes were wild-type, and the standard recording solution was SOS (115 mM NaCl, 3 mM KCl, 2 mM CaCl 2 , 5 mM MgCl 2 , 5 mM HEPES, pH 7.4), which was altered as described in the text. All chemicals were purchased from Sigma Aldrich (St. Louis, MO, USA), except D 2 O (Cambridge Isotope Labs, Andover, MA, USA). Where needed, solution exchange was performed using gravity flow. For AP experiments, oocytes were coinjected with 5 ng of complementary RNA encoding the rat Nav1.4 alpha subunit, 1 ng encoding the rat Nav beta subunit and 1 ng encoding the Shaker potassium channel. Recordings were performed 2–3 days after injection. To assess AP generation, oocytes were voltage clamped with clamp gain adjusted sufficiently low that a voltage step from −90 mV to some value around −45 mV elicited a response resembling an AP. The size of this voltage step was then reduced by ∼ 0.5 mV until no AP was fired. Traces were then acquired with and without infrared stimulation. All recordings were made at room temperature. HEK cell recordings Cultured untransfected HEK-293T cells were voltage- and current-clamped in the whole-cell configuration using the Axopatch 200B amplifier (Molecular Devices, Sunnyvale, CA, USA) at room temperature. jClamp (SciSoft Company, New Haven, CT, USA) software was used to collect and analyse the data. Recording pipets were pulled from borosilicate glass to achieve initial bath resistances averaging 3–4 MΩ, and were filled with an intracellular solution containing (mM): 140 NaCl, 2 MgCl 2 , 5 HEPES (pH 7.4). Cells were bathed during whole-cell recordings in an extracellular solution containing (mM): 140 NaCl, 2 MgCl 2 , 5 HEPES (pH 7.4); both solutions were modified as stated in the text. To measure membrane capacitance, a dual sinusoidal voltage stimulus (195.3 and 390.6 Hz with 10 mV amplitude) was applied at 0 mV, and the resulting currents were analysed using a fast Fourier transform-based admittance method [32] . Artificial lipid bilayer recordings Artificial lipid bilayers comprising PS, PC and PE (Avanti Polar Lipids, Birmingham, AL, USA) were painted on a small horizontal hole ( ∼ 300 μm in diameter) in a polyoxymethylene (delrin) partition separating two chambers. Phospholipids were dissolved in decane to a final concentration of 25 mg ml −1 , deposited near the hole, allowed to dry, then painted using air bubbles in the presence of the recording buffer (140 mM NaCl, 5 mM HEPES, pH 7.4). Bilayer quality was assessed by monitoring current responses to a voltage ramp. To alter buffer composition bathing one side of the formed bilayer, 100× concentrated solutions were carefully pipetted into the appropriate chamber. Voltage-clamp recordings were made using an Axopatch 200 A amplifier. For membrane potential recordings in the high-impedance lipid bilayers, a custom electrometric amplifier was constructed. All data were collected using in-house software. To measure membrane capacitance, sinusoidal voltage stimuli were applied at frequencies of 200–3200 Hz, and the peak-to-peak magnitudes of resulting currents (for example, Supplementary Fig. S4 ) were used to calculate changes in circuit admittance [18] . Modelling artificial bilayers as a parallel RC circuit with a very high resistance, changes in membrane capacitance were proportional to changes in admittance. All recordings were made at room temperature. Local temperature measurements Local temperature measurements were made using pipet resistance, following the method of Yao et al . [17] Pipets were filled with solution matching the extracellular recording buffer, resistance 5–10 MΩ. The tip of the pipet was positioned near the optical fibre providing infrared stimulation at a distance approximating oocyte or bilayer position. A 10-mV MΩ −1 current pulse was applied by the OC-725A amplifier to measure pipet resistance. A resistance–temperature calibration curve was obtained by applying hot solution ( ∼ 50 °C) and allowing it to cool while simultaneously recording pipet resistance and solution temperature. A linear calibration relationship was then fitted to log(resistance) versus 1/temperature (for example, Supplementary Fig. S5 ). Resistance time courses were then collected during the application of infrared pulses and converted to temperature time courses using the calibrated relationship. Statistical analysis All error bars in figures and ±values reported in the text are s.e.m. Mathematical modelling We implemented a coupled double layer model of a bilayer capacitor following the formulation of GCS theory by Genet et al [22] , with the addition of a Stern layer reflecting the size of hydrated ions in solution and the polar lipid head groups. Equations (1) and (2) relate the intrinsic and transmembrane potential-induced charges on both sides of the bilayer to potentials at each bilayer surface, corrected by the Stern potential drop on each side (described by Eqs. 3,4,5,6 below). Mathematica (Wolfram Research, Champaign, IL, USA) was used to numerically solve the full set of equations for Φ o and (Φ i − V m ) at a given temperature. Φ o and Φ i were then used to calculate a value for membrane mobile charge using an approximation of the bilayer core capacitance. Current was calculated as the derivative of this charge with respect to time. Equation variables and parameters are listed in Table 1 ; values are listed in Table 2 . The aqueous dielectric constant was taken to vary with temperature linearly between 20 °C and 60 °C. Table 1 Definitions of variables used in equations (1–6). Full size table Table 2 Values of parameters used in simulations of IR-induced currents. Full size table How to cite this article: Shapiro, M.G. et al . Infrared light excites cells by changing their electrical capacitance. Nat. Commun. 3:736 doi: 10.1038/ncomms1742 (2012).